Myosin Vb controls biogenesis of post-Golgi Rab10 carriers during axon development Polarized membrane addition is crucial for axon development and elongation during neuronal morphogenesis. This process is believed to be regulated by directed membrane trafficking of Rab10-containing post-Golgi carriers. However, the mechanisms underlying the biogenesis of these carriers remain unclear. Here, we report that Rab10 interaction with myosin Vb (MYO5B) determines the formation of Rab10 carriers and is important for axon development. Rab10 interacts with the exon D-encoded domain of MYO5B. Downregulating the expression of MYO5B (+D) or blocking its interaction with Rab10 impairs the fission of Rab10 vesicles from trans-Golgi membranes, causes a decrease in the number of Rab10 transport carriers and inhibits axon development in cultured hippocampal neurons. Furthermore, the MYO5B–Rab10 system is required for axon development of vertebrate neocortical neurons or zebrafish retinal ganglion cells in vivo . Thus, specific interaction between Rab10 and MYO5B controls the formation of Rab10 vesicles, which is required for axon development. Axon development requires asymmetric cytoskeletal dynamics as well as new membrane addition from the intracellular supply [1] , [2] , [3] , [4] . It is believed that plasmalemmal precursor vesicles (PPVs) provide the sources of lipids and proteins required for this membrane supply [3] . Recently, we have shown that Lgl1, the mammalian homolog of Drosophila tumor suppressor Lethal giant larvae, controls directional membrane insertion during neuronal polarization, by promoting membrane recruitment and activation of Rab10 (ref. 5 ). Like other vesicles, intracellular trafficking of Rab10 carriers may also need coordination of the following consecutive steps: initiation from a donor membrane, transportation along cytoskeletal tracks, and their tethering and fusion with the acceptor membrane. Indeed, different members of Rab family small GTPases are involved in trafficking, targeting and fusion of transport vesicles to acceptor compartments through distinct or shared effectors [6] , [7] , [8] . Among around 70 mammalian Rabs, Rab10 has been shown to mediate trafficking of membrane proteins to the plasmalemma in non-neuronal cells [9] . Recently, we found that Rab10 marks a type of PPV required for polarized membrane insertion during axon development [5] . Like other post-Golgi carriers, Rab10 vesicles should also derive from trans-Golgi membranes, a step that involves donor membrane deformation or budding, sorting and fission from the trans-Golgi cisternae. However, mechanisms regulating the biogenesis of Rab10 vesicles remain unknown. Myosins are generally considered as a family of motor proteins that transport cargos along actin filaments. At least 18 distinct classes of myosins have been identified and each of them exhibits particular cellular localization and functions [10] , [11] , [12] . Among them, the best characterized class is myosin V (MYO5), a family of processive molecular motor with two motor domains connected to extended necks and the globular tails that mediate association with various cargos [13] , [14] . In mammals, there are three isoforms of MYO5—MYO5A, MYO5B and MYO5C [15] , with each subjecting to alternative splicing in a tissue-specific manner [16] , [17] , [18] . A number of studies have shown roles of MYO5 in neuronal transportation, exocytosis and synaptic plasticity [19] . For example, MYO5A transports endoplasmic reticulum vesicles [20] , secretory vesicles [21] , tetanus toxin [22] or mitochondria [23] in axons and mRNA/protein complex into dendritic spines [24] . Moreover, MYO5 controls exocytosis of large dense core vesicles [25] and the recycling of AMPA-type glutamate receptors to dendritic spines [26] , [27] , [28] . Here, we find that MYO5B interacts with Rab10 residing on trans-Golgi membranes through exon D, and this interaction determines fission of post-Golgi Rab10 carriers. Blocking MYO5B interaction with Rab10 inhibits polarized membrane insertion, as well as axon development. Thus, we conclude that MYO5B controls biogenesis of Rab10 vesicles that are required for neuronal polarization and axon development. MYO5B exon D binds to GTP-bound form of Rab10 In a proteomic screening based on mass spectrometry analysis (MS) for Rab10 effectors, we identified MYO5B from rat brain homogenates as one of the interesting hits (data not shown), confirming that MYO5 interacts with Rab10 (ref. 18 ). Immunoprecipitation (IP) of cultured rat cortical neurons with anti-MYO5B antibody caused co-IP of Rab10, indicating the association between Rab10 and MYO5B in the brain ( Fig. 1a ). Given that exon D of MYO5 is required for its interaction with Rab10 (ref. 18 ), we determined MYO5 splicing isoforms in the brain. We found that two isoforms of MYO5B with and without exon D are expressed in the rat brain, whereas MYO5A lacks exon D and MYO5C is not expressed in the brain ( Fig. 1b ). Notably, the sequence of exon D is conserved among different species ( Fig. 1c ). We confirmed the interaction between Rab10 and MYO5B isoforms co-expressed in HEK 293 cells. 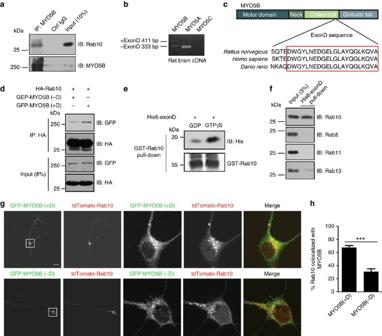Figure 1: Rab10 interacts with MYO5B via exon D. (a) Lysates of cultured cortical neurons were subject to IP with MYO5B antibody or control IgG, followed by IB with antibodies against Rab10 or MYO5B. (b) Transcription of MYO5A and MYO5B isoforms in the P0 rat brain. The amplified 411 bp and 333 bp bands in RT-PCR represent MYO5B isoforms with (+) and without (−) exon D, respectively. (c) Exon D of MYO5B is conserved among different species indicated by the amino acids alignment. (d) Cell lysates of HEK 293 cells transfected with HA-Rab10 and GFP-MYO5B without or with exon D were subject to IP with HA antibody, and then IB with HA or GFP antibody. (e) GST-Rab10 immobilized on glutathione Sepharose beads was preloaded with GTPγS or GDP, and then incubated with purified His6-exon D. Bound proteins were subject to IB with His antibody. (f) His6-ExonD immobilized on Ni-NTA agarose was incubated with lysates of cultured cortical neurons. Beads-associated proteins were determined by IB with indicated antibodies. (g) Cultured hippocampal neurons were co-transfected with TD-Rab10 and GFP-MYO5B (+D) or MYO5B (−D). At DIV3, transfected neurons were imaged to determine the localization of Rab10 and MYO5B isoforms. The enlarged areas show perinuclear regions with a large fraction of Rab10 colocalized with MYO5B (+D), compared to a lesser extent with MYO5B (−D). (h) Quantification for the proportion of Rab10 vesicles colocalized with MYO5B vesicles (see detailed information in Methods). Data are shown as mean±s.e.m. At least 20 neurons from each group were analyzed. ***P<0.001, Student’st-test. Scale bar=20 μm. As shown in Figure 1d , hemagglutinin (HA)-tagged Rab10 was co-precipitated strongly with GFP-tagged MYO5B (+D), and weakly with MYO5B (−D). The weak association between Rab10 and MYO5B (−D) might be mediated indirectly by common effectors shared by Rab10 and other Rabs, such as Rab11 Family Interacting Protein 2 (FIP2) [18] , [29] . To determine whether exon D itself is able to bind Rab10, we used beads coupled with glutathione S-transferase (GST)–Rab10 fusion protein to pull-down affinity-purified hexahistidine (His6)-tagged exon D. As shown in Fig. 1e , exon D preferentially binds to Rab10 preloaded with GTPγS, suggesting the direct interaction between Rab10 and exon D and that MYO5B might be an effector of Rab10. There was no direct interaction between MYO5B exon D and Rab8, Rab11 or Rab13 ( Fig. 1f ), indicating the specificity of exon D interaction with Rab10. When expressed in fibroblasts, tdTomato-tagged Rab10 (TD-Rab10) exhibited vesicular localization and was largely colocalized with GFP-tagged MYO5B (+D) ( Supplementary Fig. S1a,b ). However, the percentage of Rab10 colocalized with GFP-MYO5B (−D) was significantly decreased ( Supplementary Fig. S1a,b ), in line with the notion that exon D is required for the interaction with Rab10 (ref. 18 ). Figure 1: Rab10 interacts with MYO5B via exon D. ( a ) Lysates of cultured cortical neurons were subject to IP with MYO5B antibody or control IgG, followed by IB with antibodies against Rab10 or MYO5B. ( b ) Transcription of MYO5A and MYO5B isoforms in the P0 rat brain. The amplified 411 bp and 333 bp bands in RT-PCR represent MYO5B isoforms with (+) and without (−) exon D, respectively. ( c ) Exon D of MYO5B is conserved among different species indicated by the amino acids alignment. ( d ) Cell lysates of HEK 293 cells transfected with HA-Rab10 and GFP-MYO5B without or with exon D were subject to IP with HA antibody, and then IB with HA or GFP antibody. ( e ) GST-Rab10 immobilized on glutathione Sepharose beads was preloaded with GTPγS or GDP, and then incubated with purified His6-exon D. Bound proteins were subject to IB with His antibody. ( f ) His6-ExonD immobilized on Ni-NTA agarose was incubated with lysates of cultured cortical neurons. Beads-associated proteins were determined by IB with indicated antibodies. ( g ) Cultured hippocampal neurons were co-transfected with TD-Rab10 and GFP-MYO5B (+D) or MYO5B (−D). At DIV3, transfected neurons were imaged to determine the localization of Rab10 and MYO5B isoforms. The enlarged areas show perinuclear regions with a large fraction of Rab10 colocalized with MYO5B (+D), compared to a lesser extent with MYO5B (−D). ( h ) Quantification for the proportion of Rab10 vesicles colocalized with MYO5B vesicles (see detailed information in Methods). Data are shown as mean±s.e.m. At least 20 neurons from each group were analyzed. *** P <0.001, Student’s t -test. Scale bar=20 μm. Full size image MYO5B–Rab10 interaction determines neuronal polarization Isolated hippocampal neurons from rat embryos undergo spontaneous axon development in culture [30] , [31] . Shortly after adherence to the culture substratum, these neurons extend several short neurites with similar length (Stage 2). After 24–36 h, however, one of the neurites exhibits accelerated growth and later becomes the axon (Stage 3). The transition from Stage 2 to Stage 3 is a critical period for axon specification, and this process needs asymmetric membrane supply that involves Rab10-positive vesicles [5] . Interestingly, we found that TD-Rab10 was largely colocalized with GFP-MYO5B (+D) in the somatic region, especially in perinuclear areas proximal to axon initiation sites in polarized hippocampal neurons ( Fig. 1g ). Notably, much lesser Rab10 was colocalized with MYO5B (−D) ( Fig. 1g ), indicating that exon D domain is required for the interaction with Rab10 in neurons. To determine roles of MYO5B isoforms in axon development, we downregulated the expression of MYO5B (+D) by using small interfering RNAs (siRNAs). Because of the lack of antibody that can distinguish MYO5B (+D) and MYO5B (−D), we chose to test the efficacy of siRNAs by measuring levels of mRNAs of respective MYO5B isoforms using reverse transcription PCR (RT-PCR). As shown in Fig. 2a , the expression of mRNA of endogenous MYO5B (+D), but not that of MYO5B (−D), was suppressed by the siRNA specifically targeted against exon D of MYO5B (siMYO5B) in cultured cortical neurons. We found that transfection of cultured hippocampal neurons before cell plating with siMYO5B plasmids impaired axon formation ( Fig. 2b ). The effect of siMYO5B on axon formation was reflected from the reduced percentage of neurons with single axons, which positively stained with SMI-312, as compared to cultures transfected with plasmid encoding scrambled sequence (siScramble) ( Fig. 2b ). The defect in axon formation of siMYO5B neurons was markedly prevented by co-transfection with siRNA-resistant form of MYO5B (+D), hereafter referred to as MYO5B (+D)-Res, but not by MYO5B (−D) ( Fig. 2b ). This result indicates the importance of exon D domain for the function of MYO5B in axon development. To determine whether the motor activity of MYO5B is required for axon development, we generated mutated forms of MYO5B in the background of MYO5B (+D)-Res. Both the S217A mutation in switch I and the G440A/E442A double mutations in switch II inhibit ATP hydrolysis activity, and thus exhibit reduced run length on actin filaments [32] , [33] , [34] . Interestingly, neither S217A nor G440A/E442A could rescue axon developmental defect caused by siMYO5B ( Fig. 2b ). Thus, the motor activity of MYO5B is required for its function in regulating axon development. 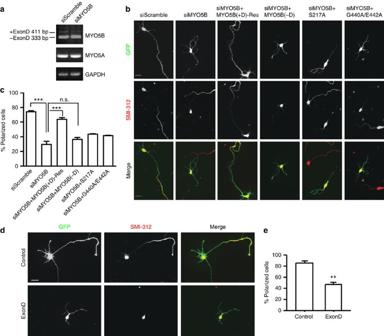Figure 2: MYO5B interaction with Rab10 is required for neuronal polarization of cultured hippocampal neurons. (a) Cultured cortical neurons transfected with siRNA against MYO5B exon D or scrambled sequence were analyzed by RT-PCR for the expression of MYO5B isoforms. Note the effective down-regulation of MYO5B (+D), but not MYO5B (−D), MYO5A, or GAPDH. (b) Isolated hippocampal neurons were transfected with constructs encoding siRNA against scrambled sequence or MYO5B, either alone or together with indicated MYO5B constructs. At DIV3, cultures were stained with axonal marker SMI-312 antibody. Neurons with one single axon were considered as normally polarized. (c) Quantification for the percentage of neurons with normal polarity. Data are shown as mean±s.e.m from three independent experiments. At least 50 neurons from each group were analyzed in each experiment. **P<0.01, ***P<0.001, one-way ANOVA. Scale bar=20 μm. (d) Cultured hippocampal neurons transfected with GFP or GFP-exon D were stained with SMI-312 antibody at DIV3. (e) Quantification for neuronal polarity. At least 50 neurons from each group were analyzed. Data are shown as mean±s.e.m. **P<0.01, Student’st-test. Scale bar=20 μm. Figure 2: MYO5B interaction with Rab10 is required for neuronal polarization of cultured hippocampal neurons. ( a ) Cultured cortical neurons transfected with siRNA against MYO5B exon D or scrambled sequence were analyzed by RT-PCR for the expression of MYO5B isoforms. Note the effective down-regulation of MYO5B (+D), but not MYO5B (−D), MYO5A, or GAPDH. ( b ) Isolated hippocampal neurons were transfected with constructs encoding siRNA against scrambled sequence or MYO5B, either alone or together with indicated MYO5B constructs. At DIV3, cultures were stained with axonal marker SMI-312 antibody. Neurons with one single axon were considered as normally polarized. ( c ) Quantification for the percentage of neurons with normal polarity. Data are shown as mean±s.e.m from three independent experiments. At least 50 neurons from each group were analyzed in each experiment. ** P <0.01, *** P <0.001, one-way ANOVA. Scale bar=20 μm. ( d ) Cultured hippocampal neurons transfected with GFP or GFP-exon D were stained with SMI-312 antibody at DIV3. ( e ) Quantification for neuronal polarity. At least 50 neurons from each group were analyzed. Data are shown as mean±s.e.m. ** P <0.01, Student’s t -test. Scale bar=20 μm. Full size image To further determine the role of Rab10–MYO5B system in axon development, cultured hippocampal neurons were transfected with GFP-exon D plasmid to block the interaction between endogenous Rab10 and MYO5B (+D). Similar to the effect of siMYO5B, overexpression of exon D also caused a decrease in the percentage of polarized cells with single axon ( Fig. 2d ). Thus, MYO5B interaction with Rab10 determines neuronal polarization in culture hippocampal neurons. Rab10–MYO5B interaction determines Rab10 vesicle formation How does the interaction between Rab10 and MYO5B affect axon development? A reasonable hypothesis is that MYO5B may determine transport of Rab10 vesicles required for directional membrane insertion. However, Rab10 vesicles were not well colocalized with MYO5B (+D) in the shafts or growth cones of neurites or axons of cultured hippocampal neurons ( Fig. 1g ). In contrast, Rab10 and MYO5B (+D) were largely colocalized in the perinuclear regions ( Fig. 1g ), which were enriched with trans-Golgi network signal TGN38 ( Supplementary Fig. S2a ). Notably, immuno-electron microscopy (EM) showed that Rab10 and IGFR-β, the receptor for insulin-like growth factor, which is believed to be a marker for PPV [35] , were observed in the Golgi or perinuclear membrane structures of the rat cortex ( Supplementary Fig. S2b,c ). These findings prompted us to determine the role of Rab10–MYO5B system in the biogenesis of post-Golgi Rab10 carriers. We found that in cultured hippocampal neurons at DIV1, TD-Rab10 exhibited vesicular distribution and a pool of Rab10 was colocalized with TGN38 ( Fig. 3a ; top rows). Interestingly, when MYO5B (+D) was downregulated, the number of Rab10 vesicles was markedly reduced ( Fig. 3b ), and more Rab10 was accumulated at TGN regions, as indicated by increased colocalization between Rab10 and TGN38 ( Fig. 3c ). Of note, downregulation of MYO5B had no apparent effect on the distribution of TGN38 ( Fig. 3e ). The decrease in the number of Rab10 vesicles and increase in the accumulation at TGN were prevented by co-expression of MYO5B (+D)-Res, but not mutants with impaired motor activity, or MYO5B (−D) ( Fig. 3b–d ). Thus, the motor activity and exon D domain of MYO5B are crucial for the formation of post-Golgi Rab10 carriers. 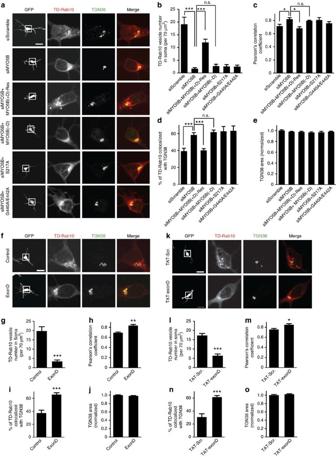Figure 3: Rab10 interaction with MYO5B determines formation of Rab10 vesicles in developing neurons. (a–e) Isolated hippocampal neurons were transfected with TD-Rab10 together with control or MYO5B siRNA, without or with indicated constructs. At DIV1, cultures were stained with TGN38 antibody (a). Numbers of TD-Rab10 vesicles in the soma were quantified (b). The Pearson’s correlation coefficient (c) and percentage voxels of TD-Rab10 colocalized with TGN38 (d) were analyzed using Image J (see detailed information in Methods). TGN38 area in the soma was quantified and normalized with values from control group set as 1 (e). Data are shown as mean±s.e.m from three experiments. At least 15 neurons at each group were analyzed. *P<0.05, ***P<0.001; n.s., no significant difference; One-way ANOVA. Scale bar=20 μm. (f–j) Hippocampal neurons transfected with TD-Rab10 together with GFP-exon D or GFP were stained with TGN38 at DIV1 (f). Number of TD-Rab10 vesicles in the soma was quantified (g). The Pearson’s correlation coefficient (h) and percentage voxels of TD-Rab10 colocalized with TGN38 (i) were analyzed using Image J. TGN38 area in the soma was quantified and normalized with values from control group set as 1 (j). **P<0.01, ***P<0.001. Student’st-test. Scale bar=20 μm. (k–o) DIV1 hippocampal neurons transfected with TD-Rab10 were treated with 40 μM TAT-exonD or same amount of TAT-scramble peptides for 1.5 h, followed by staining with TGN38 antibody (k) and the quantification for the number of TD-Rab10 vesicles (l), the Pearson’s correlation coefficient (m), percentage voxels of TD-Rab10 colocalized with TGN38 (n), and TGN38 area (o). Data are shown as mean±s.e.m. *P<0.05, ***P<0.001, Student’st-test. Scale bar=20 μm. Figure 3: Rab10 interaction with MYO5B determines formation of Rab10 vesicles in developing neurons. ( a – e ) Isolated hippocampal neurons were transfected with TD-Rab10 together with control or MYO5B siRNA, without or with indicated constructs. At DIV1, cultures were stained with TGN38 antibody ( a ). Numbers of TD-Rab10 vesicles in the soma were quantified ( b ). The Pearson’s correlation coefficient ( c ) and percentage voxels of TD-Rab10 colocalized with TGN38 ( d ) were analyzed using Image J (see detailed information in Methods). TGN38 area in the soma was quantified and normalized with values from control group set as 1 ( e ). Data are shown as mean±s.e.m from three experiments. At least 15 neurons at each group were analyzed. * P <0.05, *** P <0.001; n.s., no significant difference; One-way ANOVA. Scale bar=20 μm. ( f – j ) Hippocampal neurons transfected with TD-Rab10 together with GFP-exon D or GFP were stained with TGN38 at DIV1 ( f ). Number of TD-Rab10 vesicles in the soma was quantified ( g ). The Pearson’s correlation coefficient ( h ) and percentage voxels of TD-Rab10 colocalized with TGN38 ( i ) were analyzed using Image J. TGN38 area in the soma was quantified and normalized with values from control group set as 1 ( j ). ** P <0.01, *** P <0.001. Student’s t -test. Scale bar=20 μm. ( k – o ) DIV1 hippocampal neurons transfected with TD-Rab10 were treated with 40 μM TAT-exonD or same amount of TAT-scramble peptides for 1.5 h, followed by staining with TGN38 antibody ( k ) and the quantification for the number of TD-Rab10 vesicles ( l ), the Pearson’s correlation coefficient ( m ), percentage voxels of TD-Rab10 colocalized with TGN38 ( n ), and TGN38 area ( o ). Data are shown as mean±s.e.m. * P <0.05, *** P <0.001, Student’s t -test. Scale bar=20 μm. Full size image Next, the role of Rab10–MYO5B interaction in the formation of Rab10 vesicles was determined by overexpressing exon D or treating cultured neurons with cell permeable peptides composed of the TAT sequence derived from the trans-activator of transcription of human immunodeficiency virus and the exon D or scrambled sequence. Similar to the effect of siMYO5B, overexpression of exon D also caused a marked reduction in the number of Rab10 vesicles ( Fig. 3f ) and increased accumulation of Rab10 in TGN regions ( Fig. 3h ), without affecting TGN ( Fig. 3j ). Moreover, treatment with TAT-exonD (40 μM, 1.5 h), which was able to acutely disrupt the association between Rab10 and MYO5B ( Supplementary Fig. S1c,d ), also caused similar effects on patterns of Rab10 distribution ( Fig. 3k–o ). We also evaluated localization of endogenous Rab10 by immunostaining after above treatments and found similar tendency ( Supplementary Fig. S3a–f ). These results suggest that MYO5B and its interaction with Rab10 are important for the formation of Rab10 vesicles, whose directional membrane insertion is critical for neuronal polarization. The failure in the formation of Rab10 vesicles in siMYO5B or exon D neurons might perturb polarized distribution of Rab10. Using Tuj1 (β-Tubulin III) as a marker for neurite volume, we found that Rab10 intensity was indeed significantly higher in the axon than in other neurites of cultured hippocampal neurons at DIV 3 ( Supplementary Fig. S4a–d , see red arrow heads). However, in siMYO5B or exon D-transfected neurons, this polarized distribution of Rab10 was impaired, with Rab10 signals evenly distributed to all neurites ( Supplementary Fig. S4c,d ). The impairment in polarized distribution of Rab10 caused by siMYO5B was prevented by co-expression of MYO5B (+D)-Res, but not MYO5B (−D) ( Supplementary Fig. S4a,c ). The failure in the formation of Rab10 vesicles may also lead to impairment in polarized membrane insertion of PPV-associated membrane proteins to the plasma membrane. What types of membrane proteins are contained in Rab10 vesicles? Immune-EM analysis showed that in the P0 rat brain sections covering the regions of callosal commissure, the pleiomorphic Rab10 vesicles were co-labeled by IGFR, TrkB or VAMP4 ( Fig. 4a ). Interestingly, in cultured hippocampal neurons transfected with siMYO5B or exon D, IGFR failed to be localized to the cell surface ( Fig. 4b ), although total levels of IGFR remained unchanged ( Supplementary Fig. S5a ). In contrast, in control cells transfected with siScramble and vehicle plasmids, surface or total IGFR was found in distal regions of axons ( Fig. 4b and Supplementary Fig. S5a , see red arrowheads). We also found marked accumulation of IGFR in the cell body of siMYO5B-transfected cells ( Supplementary Fig. S5b,c , see red arrows), suggesting the failure to exit Golgi. Thus, MYO5B and its interaction with Rab10 have an important role in the formation of post-Golgi carriers, which exhibit polarized distribution during axon development. 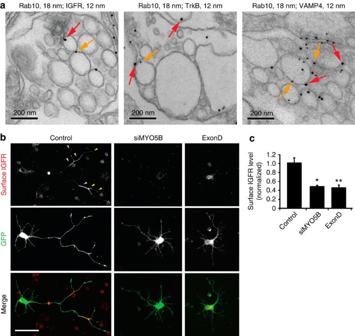Figure 4: Rab10 regulates surface expression of axonal membrane proteins. (a) Immuno-EM analysis for subcellular localization of indicated proteins and Rab10 in the corpus callosum regions from P0 rat brain. Red arrows indicate immunogold particles (18 nm) for Rab10 signals associated with PPV-like vesicles which were also marked by IGFR, TrkB or VAMP4 (yellow arrows, 12 nm). Scale bars=200 nm. (b) DIV2 hippocampal neurons transfected with vehicle plasmid or that encodes siMYO5B or exon D were live-stained with IGFR antibody without penetration. Co-expressed GFP was used to normalize neurite volumes. Note the polarized surface localization of IGFR in control cells was lost in siMYO5B or exon D neurons. Scale bar=50 μm. (c) Quantification for the surface IGFR signals in various groups. Data are presented as mean±s.e.m, with value from control group normalized as 1. *P<0.05, **P<0.01, Student’st-test (n=5 for each group). Figure 4: Rab10 regulates surface expression of axonal membrane proteins. ( a ) Immuno-EM analysis for subcellular localization of indicated proteins and Rab10 in the corpus callosum regions from P0 rat brain. Red arrows indicate immunogold particles (18 nm) for Rab10 signals associated with PPV-like vesicles which were also marked by IGFR, TrkB or VAMP4 (yellow arrows, 12 nm). Scale bars=200 nm. ( b ) DIV2 hippocampal neurons transfected with vehicle plasmid or that encodes siMYO5B or exon D were live-stained with IGFR antibody without penetration. Co-expressed GFP was used to normalize neurite volumes. Note the polarized surface localization of IGFR in control cells was lost in siMYO5B or exon D neurons. Scale bar=50 μm. ( c ) Quantification for the surface IGFR signals in various groups. Data are presented as mean±s.e.m, with value from control group normalized as 1. * P <0.05, ** P <0.01, Student’s t -test ( n =5 for each group). Full size image MYO5B–Rab10 interaction determines Golgi fission of PPVs Formation of post-Golgi carrier vesicles involves remodeling, elongation and fission at the trans-Golgi network. Next, we determined which specific step MYO5B participates in regulating the formation of Rab10 vesicles. We found that endogenous vesicular Rab10 distributed in regions from perinuclear to cell periphery of fibroblasts ( Fig. 5a ). A pool of Rab10 was colocalized with TGN38 in perinuclear regions ( Fig. 5a ). We followed the dynamics of the Rab10-labeled vesicles using time-lapse microscopy, under the conditions without or with MYO5B downregulation. In control cells transfected with TD-Rab10 and vehicle plasmids, we often observed the dynamic process for the formation of Rab10 vesicles, which are composed of the following consecutive steps—membrane extension from the perinuclear to form a tubular structure, fission of tubules to form carrier vesicles, followed by transportation of the carrier vesicle to the cell periphery and retraction of the original tubule ( Fig. 5b , top row, and ,Supplementary Movie 1). Interestingly, when expression of MYO5B (+D) was downregulated, more tubular structures emerged from perinuclear regions. Usually, these tubules persisted for several minutes without fission during the observation periods (Supplementary Movie 2 and Fig. 5b , the second row from top). As a result, the static number of TD-Rab10 tubules was increased in siMYO5B cells, compared with control cells transfected with siScramble and vehicle plasmids ( Fig. 5c ). Notably, siMYO5B transfection also caused an increase in the percentage of cells exhibiting TD-Rab10 tubules in cultured cortical neurons ( Supplementary Fig. S6a,b , see also Supplementary Movie 5 and 6) and endogenous Rab10 tubules in fibroblasts ( Supplementary Fig. S7a,c ). Sometimes, these unfissioned Rab10 attached together to form big vacuoles ( Supplementary Fig. S6 and Supplementary Movie 6), and this phenomena was never seen in control cells. Thus, MYO5B (+D) is essential for the formation of Rab10 vesicles, most likely at the step of membrane fission, rather than the steps of deformation or elongation of TGN membranes. In line with the role of MYO5B (+D) in the fission of Rab10 vesicles from TGN, the number of Rab10-postive vesicles undergoing transportation after fission was decreased in siMYO5B cells ( Fig. 5c ). Notably, either the increase in tubular structures or the decrease in transport vesicles caused by siMYO5B was largely prevented by expression of MYO5B (+D)-Res, but not MYO5B (−D) ( Fig. 5b–e , also see Supplementary Movies 3, 4, 7 and 8, Supplementary Figs S6, and S7c ). Thus, exon D domain of MYO5B is essential for the sorting of Rab10 vesicles from the TGN membranes. 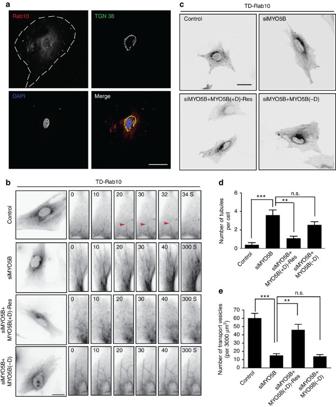Figure 5: MYO5B exon D is required for the fission of Rab10 vesicles from TGN. (a) Rat fibroblasts were stained with antibodies against Rab10 and TGN38, with DAPI labeling nucleus. Note the perinuclear and periphery localization of Rab10 signals. (b) Time-lapse photography showing the dynamic process for the formation of Rab10 vesicles in fibroblasts transfected with TD-Rab10 together with indicated constructs. Note a typical fission event of Rab10 vesicle from perinuclear TGN region (red arrowhead). (c) Representative images showing TD-Rab10 patterns in fibroblasts transfected with indicated constructs. Scale bar=20 μm. (d) Quantification for the number of tubule-like structures in each cell with various transfections. (e) Quantification for Rab10 vesicles normalized by cell area. Data are presented as mean±s.e.m. At least 15 cells at each group were analyzed. **P<0.01; ***P<0.001; n.s., no significant difference; One-way ANOVA. Figure 5: MYO5B exon D is required for the fission of Rab10 vesicles from TGN. ( a ) Rat fibroblasts were stained with antibodies against Rab10 and TGN38, with DAPI labeling nucleus. Note the perinuclear and periphery localization of Rab10 signals. ( b ) Time-lapse photography showing the dynamic process for the formation of Rab10 vesicles in fibroblasts transfected with TD-Rab10 together with indicated constructs. Note a typical fission event of Rab10 vesicle from perinuclear TGN region (red arrowhead). ( c ) Representative images showing TD-Rab10 patterns in fibroblasts transfected with indicated constructs. Scale bar=20 μm. ( d ) Quantification for the number of tubule-like structures in each cell with various transfections. ( e ) Quantification for Rab10 vesicles normalized by cell area. Data are presented as mean±s.e.m. At least 15 cells at each group were analyzed. ** P <0.01; *** P <0.001; n.s., no significant difference; One-way ANOVA. Full size image Similar to the effect of siMYO5B, overexpression of exon D caused appearance of tubular structures of endogenous or TD-Rab10 in fibroblasts ( Fig. 6a and Supplementary Fig. S7 ) or neurons ( Supplementary Fig. S6 and Supplementary Movie 9). The fission defect resulting from exon D overexpression was also reflected from increased number of TD-Rab10 tubules ( Fig. 6b ), percentage of cells with endogenous Rab10 tubules ( Supplementary Fig. S7b,d ), percentage of cortical neurons with TD-Rab10 tubules ( Supplementary Fig. S6 and Supplementary Movie 9) and decreased number of Rab10 carrier vesicles ( Fig. 6c ). Treatment with TAT-exonD also caused an increase in the number of tubules and a decrease in Rab10 vesicles, in a dose-dependent manner ( Fig. 6d–f ). Thus, the MYO5B–Rab10 interaction have an important role in the fission of deformed and elongated membrane structures of the Golgi apparatus. 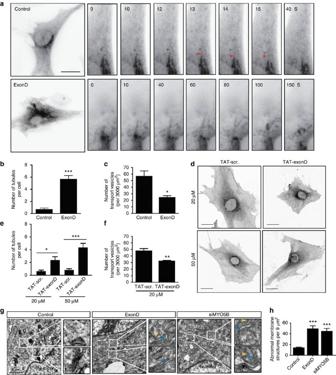Figure 6: MYO5B interaction with Rab10 determines fission of PPVs at the TGN. (a) Rat fibroblasts were transfected with TD-Rab10 together with vehicle or exon D plasmids. Time-lapse imaging shows a fission event in control cells (red arrowhead) and the persistence of a tubule-like structure that was finally collapsed in exon D cells. Scale bar=20 μm. (b,c) Quantification for the number of tubules (b) and vesicles (c). Data are shown as mean±s.e.m. At least 15 cells at each group were analyzed. *P<0.05, ***P<0.001, Student’st-test. (d–f) Fibroblasts transfected with TD-Rab10 were treated for 1.5 h with indicated amounts of TAT-exon D or scrambled peptides. The static number of tubules (e) and vesicles (f) were quantified. Data are shown as mean±s.e.m. At least 15 cells at each group were analyzed. *P<0.05, **P<0.01, ***P<0.001, Student’st-test. Scale bar=20 μm. (g) Fibroblast transfected with vehicle (control) or plasmids encoding exon D or siMYO5B were subject to EM analysis. Note the normal Golgi structure in control cell and the appearance of many tubule-like structures with heterogeneous shapes and sizes (blue arrows) in exon D or siMYO5B cells. Cross sections of tubules exhibit vesicle-like morphology (yellow arrowheads). Scale bars=500 nm. (h) Quantification for the number of abnormal membrane structures, including tubules, cross sections of tubules or accumulated vesicles per 9 μm2perinuclear region. Data are shown as mean±s.e.m. ***P<0.001, Student’st-test, at least 20 cells at each group were analyzed. Figure 6: MYO5B interaction with Rab10 determines fission of PPVs at the TGN. ( a ) Rat fibroblasts were transfected with TD-Rab10 together with vehicle or exon D plasmids. Time-lapse imaging shows a fission event in control cells (red arrowhead) and the persistence of a tubule-like structure that was finally collapsed in exon D cells. Scale bar=20 μm. ( b , c ) Quantification for the number of tubules ( b ) and vesicles ( c ). Data are shown as mean±s.e.m. At least 15 cells at each group were analyzed. * P <0.05, *** P <0.001, Student’s t -test. ( d – f ) Fibroblasts transfected with TD-Rab10 were treated for 1.5 h with indicated amounts of TAT-exon D or scrambled peptides. The static number of tubules ( e ) and vesicles ( f ) were quantified. Data are shown as mean±s.e.m. At least 15 cells at each group were analyzed. * P <0.05, ** P <0.01, *** P <0.001, Student’s t -test. Scale bar=20 μm. ( g ) Fibroblast transfected with vehicle (control) or plasmids encoding exon D or siMYO5B were subject to EM analysis. Note the normal Golgi structure in control cell and the appearance of many tubule-like structures with heterogeneous shapes and sizes (blue arrows) in exon D or siMYO5B cells. Cross sections of tubules exhibit vesicle-like morphology (yellow arrowheads). Scale bars=500 nm. ( h ) Quantification for the number of abnormal membrane structures, including tubules, cross sections of tubules or accumulated vesicles per 9 μm 2 perinuclear region. Data are shown as mean±s.e.m. *** P <0.001, Student’s t -test, at least 20 cells at each group were analyzed. Full size image Next, we analyzed ultrastructural changes in the fibroblasts transfected with exon D or siMYO5B by electroporation, which resulted in the transfection of almost all the cells. ( Supplementary Fig. S8 ). EM analysis showed that siMYO5B or exon D transfection caused abnormal accumulation of tubular or vesicular structures with heterogeneous shapes and sizes in perinuclear or periphery cell regions ( Fig. 6g , see tubules indicated by blue arrows). Some vesicular structures might be the cross sections of tubules. Thus, MYO5B determines biogenesis of Rab10 transport vesicles through the interaction with Rab10. MYO5B–Rab10 system in axon development of cortical neurons We next determined the physiological role of this regulatory mechanism in vivo . For this purpose, E16.5 rat embryos were subjected to in utero electroporation with combinations of siRNA or expression plasmids together with pCAG-EYFP to label cortical neural precursors, and then at P0, differentiation of transfected cells was determined by staining with antibodies recognizing newborn neurons at different stages and staining with GFP antibody for cell morphology. We found that in control animals that had been transfected with scrambled siRNA, transfected cortical neurons extended contralateral projecting axons traversing through the intermediate zone (IZ) toward the midline ( Fig. 7a , see a1). However, such axon projection was severely affected in siMYO5B-transfected animals ( Fig. 7a , see a2), as reflected from decreased axon length index ( Fig. 7b ). The impairment in axon development caused by MYO5B downregulation was completely prevented by co-expression of MYO5B (+D)-Res ( Fig. 7a (see a3) and 7b). Same approach was used to determine the effect of exon D overexpression. Cortical neurons transfected with exon D also exhibited reduced length of the callosal axons ( Fig. 7c ). Thus, Rab10 interaction with MYO5B has a critical role in axon development of cortical neurons in vivo . 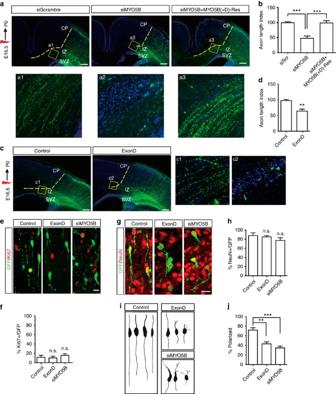Figure 7: MYO5B exon D is important for axon development of neocortical neuronsin vivo. (a,b) P0 neocortical slices from rat embryos electroporated at E16.5 with plasmids encoding scramble, siMYO5B or siMYO5B plus MYO5B (+D)-Res, together with EYFP, were analyzed for axon development. Enlarged areas (a1–a3) indicate axons coursing through the IZ. The length of these axon bundles, as sketched by yellow dashed lines which delineate the path of axonal tracts from cell bodies at the cortical plate to the front of axonal bundles in the intermediate zone (IZ), was quantified with the value from control group normalized as 100 (b). Data are presented as mean±s.e.m. ***P<0.001, Student’st-test, at least three animals were analyzed in each group. Scale bars=200 μm. (c,d) Effects of over-expression of exon D on axon development of neocortical neuronsin vivo. Enlarged areas (c1, c2) indicate axons coursing through the IZ. Data are shown as mean±s.e.m. **P<0.01, Student’st-test, at least 3 animals were analyzed for each group. Scale bars=200 μm. (e–h) P0 neocortical slices from rat embryos electroporated at E16.5 with EYFP together with indicated plasmids were co-stained with GFP and Ki67 (e) or NeuN (g) antibody. Percentage of Ki67-positive (Ki67+) or NeuN-positive (NeuN+) cells among GFP-positive cells was quantified. Data are presented as mean±s.e.m from at least 50 cells. n.s., no significant difference, Student’st-test. (i) Neurolucida tracing of individual neurons in IZ regions of P0 rats electroporated with indicated plasmids. (j) Quantification for polarized cells with a long thin descending axon. Data are presented as mean±s.e.m (n=50 for control,n=46 for siMYO5B,n=38 for Exon D). **P<0.01, ***P<0.001, Student’st-test. Figure 7: MYO5B exon D is important for axon development of neocortical neurons in vivo . ( a , b ) P0 neocortical slices from rat embryos electroporated at E16.5 with plasmids encoding scramble, siMYO5B or siMYO5B plus MYO5B (+D)-Res, together with EYFP, were analyzed for axon development. Enlarged areas (a1–a3) indicate axons coursing through the IZ. The length of these axon bundles, as sketched by yellow dashed lines which delineate the path of axonal tracts from cell bodies at the cortical plate to the front of axonal bundles in the intermediate zone (IZ), was quantified with the value from control group normalized as 100 ( b ). Data are presented as mean±s.e.m. *** P <0.001, Student’s t -test, at least three animals were analyzed in each group. Scale bars=200 μm. ( c , d ) Effects of over-expression of exon D on axon development of neocortical neurons in vivo . Enlarged areas (c1, c2) indicate axons coursing through the IZ. Data are shown as mean±s.e.m. ** P <0.01, Student’s t -test, at least 3 animals were analyzed for each group. Scale bars=200 μm. ( e – h ) P0 neocortical slices from rat embryos electroporated at E16.5 with EYFP together with indicated plasmids were co-stained with GFP and Ki67 ( e ) or NeuN ( g ) antibody. Percentage of Ki67-positive (Ki67+) or NeuN-positive (NeuN+) cells among GFP-positive cells was quantified. Data are presented as mean±s.e.m from at least 50 cells. n.s., no significant difference, Student’s t -test. ( i ) Neurolucida tracing of individual neurons in IZ regions of P0 rats electroporated with indicated plasmids. ( j ) Quantification for polarized cells with a long thin descending axon. Data are presented as mean±s.e.m ( n =50 for control, n =46 for siMYO5B, n =38 for Exon D). ** P <0.01, *** P <0.001, Student’s t -test. Full size image The observed defects in axon projection could be caused by abnormal neuronal fate determination or morphogenesis. We thus determined neuronal fate by staining with antibodies against NeuN, a marker for mature neurons, or Ki67, which labels proliferating cells. We found that the percentage of Ki67- or NeuN-positive cells among GFP-labeled transfected cells was not affected by electroporation with siMYO5B or exon D plasmids, compared with vehicle controls ( Figs. 7e–h ). Thus, MYO5B–Rab10 system does not regulate neuronal fate or cell proliferation. In addition to the effects on axon projection, newborn cortical neurons with siMYO5B or exon D expression also exhibited defects in neuronal migration, because lesser siMYO5B or exon D-electroporated cortical neurons migrated to the cortical plate (CP) ( Fig. 7a ). The migration defects were most likely caused by abnormal neuronal morphogenesis. We analyzed morphology of NeuN + neurons located in the IZ and CP regions. Interestingly, whereas most neurons of control animals exhibited polarized structure with a short leading process destined to become apical dendrite and a long trailing process destined to become axon, most neurons in animals transfected with sMYO5B or exon D failed to polarize normally ( Fig. 7i ). Thus, MYO5B–Rab10 system is needed for the polarization of neocortical neurons in vivo . MYO5B–Rab10 system in zebrafish optic nerve development Retinal ganglion cells (RGCs) provide another model for the study of axon development in vivo [36] , [37] , [38] . Upon contacts with basal laminin, the basal processes of newborn RGCs tend to form axons [39] . To determine whether the role of MYO5B–Rab10 system in axon development is conserved in other species, we analyzed axon growth of larval zebrafish RGCs after injection with morpholino oligos (MOs) against MYO5B or Rab10. As shown in Fig. 8a , RT-PCR shows that the fish MYO5B also has +D and –D isoforms, and the splice MO specific for exon D was effective in knocking down the expression of +D, but not –D isoform. The fish Rab10 has similar molecular weight with the mouse or rat homolog ( Fig. 8b ). We designed two MOs to suppress the expression of Rab10. ATG MO was designed to knockdown the translation of Rab10, and splice MO was designed based on intron–exon boundary region of Rab10 to block its splicing of transcription. Both MOs were able to suppress the expression of Rab10, in either translation or transcription levels ( Fig. 8c ). RGCs were labeled by mCherry driven by RGC precursor-specific Ath5 promoter ( Fig. 8e ) [40] . 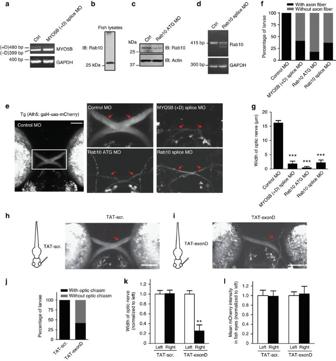Figure 8: MYO5B (+D) and Rab10 are required for axon development of zebrafish retinal ganglion cells. (a) Effect of MYO5B splice MO on the transcription of MYO5B isoforms in zebrafish larvae. Note that the expression of MYO5B (+D), but not MYO5B (−D) or GAPDH, was downregulated. (b) Immunoblot shows a single band recognized by Rab10 antibody in the homogenates of zebrafish larvae. (c) Immunoblot shows the knockdown effect of Rab10 ATG morpholino (ATG MO), using actin as a loading control. (d) RT-PCR shows the effect of Rab10 splice morpholino (splice MO) on Rab10 transcription in zebrafish larvae. The lower bands should be mis-spliced transcripts. (e) Morphology of optical chiasm labeled by mCherry in 2-dpf zebrafish larvae injected with control or MOs against MYO5B or Rab10. Scale bars=50 μm. (f,g) Quantification for the percentage of zebrafish larvae with axon fibers (f) and the width of optic nerves (g) among morphants injected with different MOs. Data are shown as mean±s.e.m. At least 10 fishes at each group from two independent experiments were analyzed. ***P<0.001 versus control MO, Student’st-test. (h,i)Tg(Ath5:gal4-uas-mCherry) transgenic larvae at 1 dpf were injected with TAT-scramble (TAT-Scr.) or TAT-exonD (10 mM, 8 nl) to the right eye and imaged at 2 dpf. Scale bar=50 μm. (j–l) Quantification for the percentage of zebrafish larvae with visible axon fibers (j), the width of optic nerves (k), and the intensity of mCherry in both eyes (l). Data are shown as mean±s.e.m. At least seven fishes at each group from two independent experiments were analyzed. **P<0.01, Pairedt-test. As shown in Fig 8e , the control fish at 2 days post-fertilization (dpf) showed normal optic chiasm that is composed of optic nerves (indicated by red arrows) traversing to the contralateral side of the brain. However, in larvae injected with MOs against MYO5B or Rab10, optic axonal tracts were severely impaired ( Fig. 8e ), as reflected from decreased percentage of larvae with visible axon tracts ( Fig. 8f ). Notably, even for those larvae with axon tracts, the width of optic axonal tracts was markedly reduced in larvae injected with MYO5B or Rab10 MOs ( Fig. 8g ). These results support the conclusion that MYO5B–Rab10 system is important for axon development in various species. Figure 8: MYO5B (+D) and Rab10 are required for axon development of zebrafish retinal ganglion cells. ( a ) Effect of MYO5B splice MO on the transcription of MYO5B isoforms in zebrafish larvae. Note that the expression of MYO5B (+D), but not MYO5B (−D) or GAPDH, was downregulated. ( b ) Immunoblot shows a single band recognized by Rab10 antibody in the homogenates of zebrafish larvae. ( c ) Immunoblot shows the knockdown effect of Rab10 ATG morpholino (ATG MO), using actin as a loading control. ( d ) RT-PCR shows the effect of Rab10 splice morpholino (splice MO) on Rab10 transcription in zebrafish larvae. The lower bands should be mis-spliced transcripts. ( e ) Morphology of optical chiasm labeled by mCherry in 2-dpf zebrafish larvae injected with control or MOs against MYO5B or Rab10. Scale bars=50 μm. ( f , g ) Quantification for the percentage of zebrafish larvae with axon fibers ( f ) and the width of optic nerves ( g ) among morphants injected with different MOs. Data are shown as mean±s.e.m. At least 10 fishes at each group from two independent experiments were analyzed. *** P <0.001 versus control MO, Student’s t -test. ( h , i ) Tg ( Ath5:gal4-uas-mCherry ) transgenic larvae at 1 dpf were injected with TAT-scramble (TAT-Scr.) or TAT-exonD (10 mM, 8 nl) to the right eye and imaged at 2 dpf. Scale bar=50 μm. ( j – l ) Quantification for the percentage of zebrafish larvae with visible axon fibers ( j ), the width of optic nerves ( k ), and the intensity of mCherry in both eyes ( l ). Data are shown as mean±s.e.m. At least seven fishes at each group from two independent experiments were analyzed. ** P <0.01, Paired t -test. Full size image To determine whether MYO5B–Rab10 interaction is important for axon development of zebrafish RGCs, TAT-exonD or scrambled peptides were injected into the right eye of Tg ( Ath5:gal4-uas-mCherry ) transgenic fish at 1 dpf, and optic nerves were observed at 2 dpf ( Fig. 8h ). Interestingly, majority of larvae injected with TAT-exonD exhibited an abnormal optic chiasm with optic nerves from the injected eye completely impaired and the uninjected eye unaffected ( Fig. 8i ). As a control, injection with TAT-scramble peptides had no effect on the formation of optic chiasm ( Fig. 8h ). We also compared the axon fibers of RGCs from two eyes of the same animal ( Fig. 8k ). We found that in the TAT-exonD-injected group, even for those larvae with optic chiasm, the width of optic axon tracts from the right eye with peptide injection was markedly decreased compared with that from the left eye without injection ( Fig. 8i (see impaired optic nerves indicated by red arrow) and 8k). This difference was not observed for animals injected with TAT-scrambled peptides ( Fig. 8h ). We next asked whether the impairment in RGC axons was due to the effect on cell health. We compared the intensity of mCherry, which was used to reflect relative number of RGCs, and found that neither injection with TAT-exonD nor TAT-scrambled peptides had caused any difference in the intensity of mCherry between the left and right eyes ( Fig. 8l ). Thus, the interaction between MYO5B and Rab10 have a critical role in the formation or maintenance of RGC axons. Axon specification and growth need the coordination between cytoskeleton dynamics and membrane trafficking [1] , [2] . Many molecules regulating cytoskeleton organization have been identified to be involved in neuronal polarization [1] , [2] . On the other hand, membrane trafficking mechanisms governing neuronal polarization are just beginning to be understood [5] , [41] , [42] . Recently, we have shown that Lgl1 has an important role in directional membrane insertion underlying axon development by activating Rab10 (ref. 5 ). Here, we have demonstrated an unexpected role of MYO5B in the biogenesis of post-Golgi Rab10 carriers and determined its role in axon development. Based on the previous study [18] and a proteomic screening, we have focused on MYO5B. We found that MYO5B binds to GTP-bound form of Rab10 via exon D, and interestingly, downregulating the expression of MYO5B (+D) or blocking its interaction with Rab10 inhibits fission of post-Golgi Rab10 carriers from the Golgi membrane. We propose a model that Rab10 residing on the Golgi is recognized by exon D domain of MYO5B, which determines sorting of Rab10 carriers. How does MYO5B promote vesicle fission at the Golgi? An attractive hypothesis is that mechanochemical properties of MYO5B may control Golgi membrane tension and deformation, thereby promote fission at the Golgi membrane. In support of this hypothesis, motor activity of MYO5B is essential for the formation of Rab10 vesicles and axon development. In line with this model, myosin Ib has been shown to be a molecular force sensor [43] , [44] , and promotes the formation of tubular-carrier precursors [45] . Another example is myosin II, which has been shown to control fission of Rab6 vesicles at the Golgi complex [46] . A number of molecules, such as dynamin 2, BARS, PKD or FAPP2, have been shown to act as fission-promoting factors [47] , [48] , [49] , [50] , [51] , [52] , [53] . It remains possible that some of these proteins may also participate in the fission of Rab10 vesicles. It is believed that axon growth requires polarized new membrane insertion [3] , [54] . In line with this notion, the Golgi apparatus is associated with the sites of axon specification [55] , [56] . It seems that several types of vesicles provide the source of the membrane precursors [5] , [41] , [57] , [58] , [59] . The possible interaction between these vesicular systems makes the dissection for the contribution of each system very difficult. In this work, we have investigated the role of post-Golgi Rab10 carriers in axon development by blocking the interaction between Rab10 and MYO5B. This study has provided evidence that Rab10 vesicle formation is indeed needed for neuronal polarization. Like other vesicles, Rab10 vesicles also need to be transported along neurite shafts and docked and fused with acceptor membranes. It is of great interest to identify motors, adapters and membrane machineries that are responsible for the trafficking of post-Golgi Rab10 carriers at various steps. Reagents Beads used for affinity purification were from GE (Glutathione-sepharose), Roche (protein A or protein G agarose) or Qiagen (Ni-NTA). Antibodies used for immunostaining (IS), immunoblotting (IB), or immune-electron microscopy (EM) were from Protein Tech Group (Rab10, 1:200 for IS or 1:300 for IB), Santa Cruz (GFP, 1:500 for IB; MYO5B, 1:200 for IB), Sigma (HA, 1:5,000 for IB; Actin, 1:5,000 for IB), Abcam (His, 1:1000 for IB, VAMP4, 1:100 for EM), Abmart (GFP, 1:2,000 for IB; Rab10, 1:200 for EM), Invitrogen (GFP, 1:1,000 for IS), Covance (SMI-312, Tuj1, 1:1,000 for IS), KangChen (GAPDH, 1:5,000 for IB), BD (Rab8, 1: 500 for IB; TGN38, 1:300 for IS), Upstate (Rab11, 1:500 for IB), Millipore (TrkB, Rab13, 1:500 for IB) or Cell signaling (IGFR-β, 1:300 for IS, 1:100 for EM). Alexa 488-, Alexa 555- or Alexa 647-conjugated secondary antibodies (1:2000 for IS) were from Invitrogen. HRP-conjugated secondary antibodies (1:4,000 for IB) were from Millipore. TAT-exon D or scrambled peptides were synthesized by GL Biochem (Shanghai) with the following sequences of amino acids: TAT-exonD, N′-YGRKKRRQRRRGSQTEDWGYLNEDGELGLAYQGLKQVA-C′; TAT-scramble, N′-YGRKKRRQRRRGLWAGLDNEAQSKTEQVYQGELGYTGL-C′. MOs were purchased from Gene Tools (Philomath, OR), with following sequences: MYO5B splice MO, 5′-GCTTTACTGCCATCCGAGTGCAAGA-3′; Rab10 ATG MO, 5′-ATAGGTCTTCTTCGCCATCTGAGCT-3′; Rab10 splice MO, 5′-ATCCCTGCACAAACACAACCACAAT-3′, control MO, 5′-CCTCTTACCTCAGTTACAATTTATA-3′. Full blots or gels for images shown in main figure panels can be found in Supplementary Fig. S9 . Constructs siRNA was designed against the exon D region of rat MYO5B with following sequence: 5′-GGCTTACCAAGGCCTAAAGCA-3′. The siMYO5B or the scramble sequence (5′-GGACCAGCCGAATTAGCTACA-3′) was synthesized and subcloned into pGPU6 vector. The construct encoding HA-tagged Rab10 or GFP-tagged MYO5B was introduced in our previous studies [5] , [60] . Exon D region of MYO5B was deleted by using Quick Change Kit (Stratagene) to form the MYO5B (−D) construct. The mutants S217A and G440AE442A were made by using Quick Change Kit (Stratagene) on the base of MYO5B (+D)-Res construct. TdTomato was subcloned into the HindIII site of pKH3-Rab10 to generate TD-Rab10. Recombinant protein purification Exon D of MYO5B was subcloned into pET32a vector. His6-exon D or GST-Rab10 recombinant fusion proteins were expressed in E. coli BL21 (DE3), followed by affinity purification using Ni-NTA agarose or Glutathione-sepharose, respectively. Immunoprecipitation and pull-down assay HEK 293 cells were cultured in DMEM supplemented with 10% fetal bovine serum (FBS) and transfected by lipofectamine 2000. Cell lysates were prepared in the cold lysis buffer (50 mM Tris (pH 7.5), 150 mM NaCl, 1% Nonidet P40) with protease inhibitors cocktail (Merck). For immunoprecipitation (IP), cell lysates (0.5–1 mg of protein in a final volume of 1 ml) were incubated with respective antibodies (1–3 μg) and subsequently with 40 μl protein A or protein G agarose beads. Immunoprecipitated proteins were resolved by SDS-PAGE, followed by IB. For guanine nucleotide selective binding assay, GST-Rab10 (5 μg) was incubated with His6-ExonD, in the presence of either 5 μM GDP or GTPγS, respectively, for 2 h at room temperature in a buffer containing 25 mM Tris (pH 7.5), 150 mM NaCl, and 5 mM MgCl 2 . Glutathione-sepharose beads were added to the mixture, incubated for 30 min, and washed with the wash buffer (25 mM Tris (pH 7.5), 150 mM NaCl, 5 mM MgCl 2 and 100 mM EDTA) for at least three times, and followed by IB. Cell culture and imaging Rat fibroblasts were isolated from E18.5 fetal rat skin and cultured in DMEM supplemented with 10% FBS at 37 °C incubator with 5% CO 2 . Rat hippocampal neurons were prepared from E18 rat embryos and digested with 0.125% trypsin-EDTA for 20 min at 37 °C followed by trituration with pipettes in the plating medium (DMEM with 10% FBS and10% F12), and then plated onto coverslips coated with poly-D-lysine. After culturing for 24 h, media was changed with neuronal culture media (neurobasal media containing 1% glutamate and 2% B27). Fibroblasts or dissociated neurons were transfected by electroporation using the Amaxa Nucleofector device before plating. For polarity analysis, neurons were fixed and stained 72 h after plating with antibodies against axonal marker SMI-312 or neuronal marker Tuj1. The fixed and stained cultures were examined by using a Neurolucida system (Nikon). For live cells, time-lapse images were acquired at a rate of 1 frame per s with Nikon Eclipse Ti-E inverted microscope with perfect focus system, equipped with CFI Apo TIRF 100 × 1.49 N.A. oil objective (Nikon), and Cascade 512B CCD camera (Photometrics, Roper Scientific). 16-bit images were projected onto the CCD chip at a magnification of 0.16 μm per pixel. For the imaging of subcellular localization, cells were fixed and stained and the fluorescence images were taken using a 60 × Plan Apo objective (NA 1.4 oil) on the NIKON FN1 confocal microscope. For the quantification of vesicle numbers, zoom 2 × is used in the imaging with a resolution of 0.1 μm/pixel. After Z-stack projection, 8-bit images were analyzed using Image J software with threshold set from 140–256. For Rab10 vesicles, the size was set as 1–9 pixels with a resolution of 0.1 μm per pixel (~0.1–0.3 μm in diameter). For accumulated IGFR puncta, the size was set as 25–160 pixels with a resolution of 0.1 μm per pixel (~0.5–1.3 μm in diameter). For the analysis of colocalization between TD-Rab10 and TGN38, the Pearson’s correlation coefficient and % voxels of colocalization of both channels were obtained from the plugin ‘Colocalization analysis—colocalization threshold’ of Image J. Percentage of Rab10 vesicles overlapped with MYO5B vesicles was quantified to indicate colocalization between these two proteins. Electron microscopy Cells were fixed for 1 h with 2.5% glutaraldehyde in 0.1 M sodium phosphate buffer, pH 7.4, followed by post-fixation with 1% osmium tetroxide for 30 min, 3 × washes with 0.1 M PBS, dehydration in ascending ethanol series, and finally embedded in araldite over 2 days. Thin sections were stained with methanolic uranyl acetate and lead citrate for morphological examination. Sections were then observed with a Joel JEM-1230 transmission electron microscope. Brain samples from cortex or corpus callosum regions of P0 rats were fixed by 4% paraformaldehyde, 0.1% picric acid and 0.05% glutaraldehyde in 0.1 M PB for 2 h at 4 °C, then cut into 200-μm slices and incubated with 1% osmic oxide for 30 min, dehydrated and embedded in Epon 812. Polymerization was carried out at 37 °C for 12 h, 45 °C for 12 h and 60 °C for 24 h. Ultra-thin sections were cut and collected on nickel grids (200 mesh), followed by staining with primary antibodies (IGFR-β, 1:100; Rab10, 1:200; TrkB, 1:100; or VAMP4, 1:100), 10 × washes with PBS, and staining with secondary antibodies conjugated with 18 nm and 12 nm gold particles (1:50, Jackson ImmunoResearch). Finally, sections were incubated with methanolic uranyl acetate and lead citrate, and observed with a Joel JEM-1230 transmission electron microscope. In utero electroporation Rat brains at E16.5 were subject to electroporation, following the injection of mixtures of plasmid DNA in Fast Green (Amresco). Briefly, DNA mixtures containing 9 μg plasmid encoding siRNA against MYO5B or scrambled sequence, 9 μg vehicle or rescue plasmid and 3 μg pCAG-EYFP plasmid were injected into the lateral ventricle of the rat brains at E16.5, which were then subject to electroporation consisting of five square wave pulses (55 V, 100 ms) with an interval of 1 s (ECM830; BTX). Five days post electroporation, coronal cryostat sections of P0 rat cortex were immediately processed for immunostaining by a free-floating protocol. Briefly, brain slices, after treatment with 0.3% Triton X-100 and 5% goat serum in PBS for 1 h, were incubated in primary antibodies (GFP, 1:500; Ki67, 1:100; NeuN, 1:200) for 24 h at 4 °C, followed by 3 × washes with PBS, and incubation with Alexa fluorescence-conjugated secondary antibodies. Zebrafish experiments Adult zebrafish ( Danio rerio ) were maintained in the National Zebrafish Resources of China (NZRC, Shanghai, China) with an automatic fish housing system (ESEN, Beijing, China) at 28 °C. Wildtype and Tg (Ath5:gal4-uas-mCherry) larvae were raised under a 14 h–10 h light-dark cycle in 10% Hank’s solution, which consisted of (in mM): 140 NaCl, 5.4 KCl, 0.25 Na 2 HPO 4 , 0.44 KH 2 PO 4 , 1.3 CaCl 2 , 1.0 MgSO 4 and 4.2 NaHCO 3 (pH 7.2), and were treated with 0.003% 1-phenyl-2-thiourea (PTU, Sigma) to prevent pigment formation. MOs dissolved in nuclease-free water were pressure-injected into one-cell stage embryos at different doses (8 ng for MYO5B splice MO, 2 ng for Rab10 ATG MO, 4 ng for Rab10 splice MO). TAT peptides (10 mM, 8 nl) were pressure-injected into the right eye of larvae at 1 dpf and images were taken from 2-dpf larvae embedded in 1% low-melting point agarose by using Nikon FN1 confocal system with 40 × (W/IR; NA, 0.80) objective lens. All animal experiments were approved by the Animal Care and Use Committee of Institute of Neuroscience, Chinese Academy of Sciences, and in compliance with ethical regulations of Shanghai Institute of Biological Sciences, Chinese Academy of Sciences. How to cite this article: Liu, Y. et al . Myosin Vb controls biogenesis of post-Golgi Rab10 carriers during axon development. Nat. Commun. 4:2005 doi: 10.1038/ncomms3005 (2013).